Organelles maintain spindle position in plant meiosis Accurate positioning of spindles is a critical aspect of cell division as it ensures that each daughter cell contains a single nucleus. In many flowering plants, two meiotic chromosome separations occur without intervening cytokinesis, resulting in two spindles in one cell during the second division. Here we report a detailed examination of two mutants, jason ( jas ) and parallel spindle1 ( ps1 ), in which disturbed spindle position during male meiosis II results in the incorporation of previously separated chromosome groups into a single cell. Our study reveals that an organelle band provides a physical barrier between the two spindles. The loss of a single protein, JAS, from this organelle band leads to its disruption and a random movement of the spindles. JAS is largely associated with vesicles in the organelle band, revealing a role for vesicles in plant meiosis and that cytoplasmic events maintain spindle position during the chromosome division. Meiosis is a special type of cell division necessary for sexual reproduction in eukaryotes, such as fungi, plants and animals [1] . Meiosis is a reductive division that involves a single round of DNA replication followed by two rounds of chromosome division to produce four cells with half the chromosome number of the mother cell. In plants, the products of meiosis undergo mitotic divisions to form gamete-containing reproductive structures. Fusion of gametes during fertilization gives rise to a new generation. While a significant amount of work had been conducted to understand chromosome dynamics during meiosis, much less is known about events that occur in the cytoplasm. The majority of dicotyledonous plants undergo simultaneous cytokinesis during male meiosis. This means that the two rounds of chromosome separation occur without intervening cell division, resulting in the formation of two spindles in one cytoplasm [2] . Mechanisms that prevent the two spindles from interacting, and thus ensure separation of the four chromosome groups, are therefore critical. When this spindle separation is disturbed it can lead to two chromosome groups being in close proximity at the end of meiosis and subsequently being incorporated into a single cell [2] . Such a cell is termed unreduced as it contains the same chromosome content as the parent cell and will give rise to unreduced gametes. Unreduced gametes are considered to be the main route to the formation of polyploid plants that contain more than two sets of chromosomes [3] , [4] , [5] , [6] , [7] . As polyploidization is a major speciation mechanism and is associated with the breeding of many important crop species [3] , [8] , [9] , there is considerable interest in understanding the mechanisms leading to unreduced gamete formation. As the separation of spindles is achieved in the vast majority of meiocytes during the second division, it implies that there are mechanisms that actively prevent the spindles from coming into close physical proximity. The discovery of two mutants in Arabidopsis thaliana that result in spindle position defects and the production of unreduced gametes offer an exciting tool to explore this mechanism. Loss of either Parallel Spindle1 ( PS1 ) [10] or Jason ( JAS ) [11] , [12] results in altered spindle position in male meiocytes and a range of meiotic products including tetrads (four reduced cells as produced in wild type), triads (two reduced and one unreduced cell) and dyads (two unreduced cells). While the PS1 and JAS proteins are required for spindle positioning, the mechanism by which this is achieved is not known, although it is proposed that they operate in a common genetic pathway [12] . In this study, we undertook a detailed microscopic analysis of the jas and ps1 mutants during male meiosis and show that cytoplasmic organization is critical for spindle position. In jas meiocytes, organelle position is disturbed early in meiosis, and an organelle band that is normally maintained between the two spindles during the second division is disturbed before alterations in spindle position occur. A JAS–green fluorescent protein (GFP) fusion protein co-localizes with markers for the endomembrane system and is associated with endomembrane vesicles within the organelle band. Combined, these results suggest that JAS-containing vesicles are required to maintain organelle position during meiosis, and in the absence of the organelle band the two spindles are no longer physically isolated and are free to interact. Furthermore, we show that jas and ps1 mutants are phenotypically distinct, implying that JAS and PS1 affect spindle positioning through different genetic pathways. JAS maintains organelle position during male meiosis To explore the mechanisms that control spindle position in plant meiosis, we undertook a detailed microscopic analysis of wild-type and jas meiocytes during the two chromosome divisions in A. thaliana ( Fig. 1 ). We focused our attention on organelle location and on microtubule dynamics and ensured that meiocytes maintained their three-dimensional structure during the observation. We used confocal laser scanning microscopy to view 4',6-diamidino-2-phenylindole (DAPI)-stained meiocytes that were still positioned in the anther locule ( Supplementary Fig. 1 ) rather than the traditional chromosome spread technique [13] in which cells become flattened and cytoplasmic contents are disturbed. This enabled us to track the location of DAPI-stained organelles (mitochondria and plastids), as well as the chromosomes. To analyse microtubule dynamics, we used a GFP–tubulin fusion protein under the control of the UBIQUITIN14 promoter ( pUBQ14:GFP–TUA6 ) [14] , [15] . While this technique required removal of meiocytes from the anther, it allowed us to visualize microtubules in cells with minimal fixation and disturbance, which is not possible with immunolocalization techniques previously used to study microtubule location in meiocytes [10] , [12] , [16] . 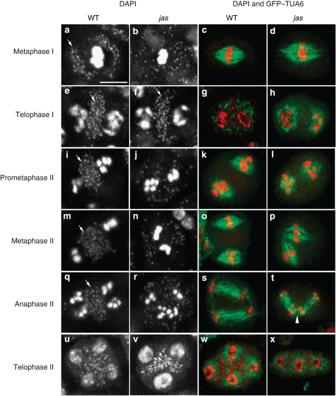Figure 1: The position of organelles is disturbed during meiosis I and II injasmeiocytes. Chromosomal and organelle DNA (fainter spots) of meiocytes in anthers stained with DAPI (left) and microtubules (green; GFP–TUA6) and DNA (red; DAPI) in meiocytes dissected from the anther (right) from wild-type (WT) andjas-3(jas) plants viewed by CLSM. Images are projection of three to five optical sections except forgthat is a single image. Stages of meiosis shown are (a–d) metaphase I, (e–h) telophase I, (i–l) prometaphase II, (m–p) metaphase II, (q–t) anaphase II and (u–x) telophase II. Arrows indicate the organelle cluster (a) or organelle band (e,f,i,m,q) and an arrowhead (t) shows where spindle positioning defects lead to the co-locating of chromosome groups. Scale bar, 10 μm. CLSM, confocal laser scanning microscopy. Figure 1: The position of organelles is disturbed during meiosis I and II in jas meiocytes. Chromosomal and organelle DNA (fainter spots) of meiocytes in anthers stained with DAPI (left) and microtubules (green; GFP–TUA6) and DNA (red; DAPI) in meiocytes dissected from the anther (right) from wild-type (WT) and jas-3 ( jas ) plants viewed by CLSM. Images are projection of three to five optical sections except for g that is a single image. Stages of meiosis shown are ( a – d ) metaphase I, ( e – h ) telophase I, ( i – l ) prometaphase II, ( m – p ) metaphase II, ( q – t ) anaphase II and ( u – x ) telophase II. Arrows indicate the organelle cluster ( a ) or organelle band ( e , f , i , m , q ) and an arrowhead ( t ) shows where spindle positioning defects lead to the co-locating of chromosome groups. Scale bar, 10 μm. CLSM, confocal laser scanning microscopy. Full size image During the first meiotic division, the chromosome structure and spindle apparatus were not noticeably disturbed in jas ( Fig. 1a–d ). There was, however, an alteration in the position of the DAPI-stained organelles. In wild-type meiocytes, the DAPI-stained organelles were tightly clustered in parts of the cytoplasm, usually in close association with the spindle, and excluded from other regions including the direct spindle location ( Fig. 1a , arrow; Supplementary Fig. 2a ). In jas , this clustering of organelles was not observed, rather the organelles were evenly spread throughout the cytoplasm ( Fig. 1b ; Supplementary Fig. 2b ). Thus, JAS is required for the clustering of organelles during the first meiotic division. Wild-type and jas meiocytes behaved in a similar manner at the completion of the first meiotic division ( Fig. 1e–h ). In both genotypes chromosomes partially decondensed and the five chromosomes formed a ring-like structure at each pole ( Fig. 1e,f ), and microtubules formed a radial array around each nucleus ( Fig. 1g,h ). Interestingly, organelle position was also similar in wild type and jas despite the differences during meiosis I, with the organelles forming a distinct band or saddle between the two nuclei ( Fig. 1e,f , arrows). This organelle band has previously been observed in a range of species, including A. thaliana , that undergo simultaneous meiotic cytokinesis [17] , [18] , [19] , [20] , [21] , [22] , [23] , [24] , [25] . As meiocytes entered the second meiotic division, the chromosomes recondensed during prometaphase II in wild type and jas ( Fig. 1i,j ). At this stage, the microtubules had invaded the nuclear space but were not yet organized into a bipolar spindle ( Fig. 1k,l ). To determine whether spindle position was already disturbed at this stage, we measured the distances between the chromosome groups at prometaphase II in meiocytes still within anthers. In wild-type and the majority of jas meiocytes, the two chromosome groups were separated by >3 μm ( Fig. 2a ). Thus, there was no major difference in the separation of the spindles as they form during prometaphase II. There was, however, a noticeable difference in the organelle location. In wild type, the central band of the organelles remained as a tight and distinct structure ( Fig. 1i , arrow; Supplementary Fig. 2e ), while in jas meiocytes the organelles were located throughout the cytoplasm, including between the chromosome groups, and were only excluded from where the spindle develops ( Fig. 1j ; Supplementary Fig. 2f ). Thus, JAS is required for the maintenance of the organelle band in meiosis II and defects in organelle position are evident early in meiosis II when the chromosome position, and therefore spindle position, is not noticeably disturbed. 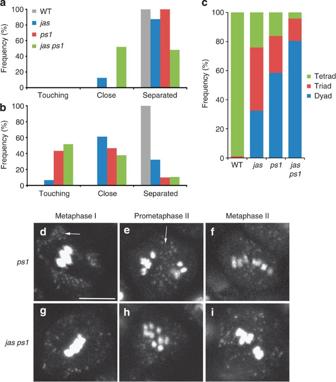Figure 2:ps1andjasare phenotypically different. The distance between the two chromosome groups at prometaphase II (a) and metaphase II (b) was measured for wild type (WT, grey;n=15 and 26),jas-3(jas, blue;n=16 and 31),ps1-1(ps1, red;n=17 and 30) and thejas-3 ps1-1double mutant (jas ps1, green;n=26 and 29). Chromosome groups were classed as touching (<0.1 μm), close (3–0.1 μm) or separated (over 3 μm apart). (c) The percentage of dyads (blue), triads (red) and tetrads (green) produced in meiosis in WT (n=831),jas-3(jas;n=1,832),ps1-1(ps;n=1,703) and thejas-3 ps1-1double mutant (jas ps;n=1,893 ) was counted in sibling plants from ajas-3+/−;ps1-1+/− parent. (d–i) Chromosomal DNA and organelles were stained with DAPI, while still in the anthers forps1-1(d–f) and thejas-3 ps1-1double mutant (g–i). Meiocytes were viewed by CLSM and images are projection of three or four optical sections. Stages of meiosis shown are (d,g) metaphase I, (e,h) prometaphase II and (f,i) metaphase II. Arrows indicate the organelle cluster (d) or organelle band (e). Scale bar, 10 μm. CLSM, confocal laser scanning microscopy. Figure 2: ps1 and jas are phenotypically different. The distance between the two chromosome groups at prometaphase II ( a ) and metaphase II ( b ) was measured for wild type (WT, grey; n =15 and 26), jas-3 ( jas , blue; n =16 and 31), ps1-1 ( ps1 , red; n =17 and 30) and the jas-3 ps1-1 double mutant ( jas ps1 , green; n =26 and 29). Chromosome groups were classed as touching (<0.1 μm), close (3–0.1 μm) or separated (over 3 μm apart). ( c ) The percentage of dyads (blue), triads (red) and tetrads (green) produced in meiosis in WT ( n =831), jas-3 ( jas ; n =1,832), ps1-1 ( ps ; n =1,703) and the jas-3 ps1-1 double mutant ( jas ps ; n =1,893 ) was counted in sibling plants from a jas-3 +/−; ps1-1 +/− parent. ( d – i ) Chromosomal DNA and organelles were stained with DAPI, while still in the anthers for ps1-1 ( d – f ) and the jas-3 ps1-1 double mutant ( g – i ). Meiocytes were viewed by CLSM and images are projection of three or four optical sections. Stages of meiosis shown are ( d , g ) metaphase I, ( e , h ) prometaphase II and ( f , i ) metaphase II. Arrows indicate the organelle cluster ( d ) or organelle band ( e ). Scale bar, 10 μm. CLSM, confocal laser scanning microscopy. Full size image During the second meiotic division, chromosomes aligned in metaphase II ( Fig. 1m–p ) and then separated in anaphase II ( Fig. 1q–t ) in both wild type and jas . In wild type, the two spindles ( Fig. 1o,s ) and chromosome groups ( Fig. 1m,q ; Fig. 2b ) remained well separated and the organelle band persisted between the two groups of chromosomes throughout the second division ( Fig. 1m,q ; Supplementary Fig. 2i ). In jas meiocytes, the chromosome groups were frequently either closer than in wild type or even touching ( Fig. 1n,r ; Fig. 2b ), which was reflected by an altered spindle position. The two spindles often had one pole of each spindle in close proximity giving a tripolar-like structure ( Fig. 1p,t ) or were close and aligned along their length ( Supplementary Fig. 3d,e ). In some jas meiocytes, chromosome separation ( Fig. 2b ) and spindle position ( Supplementary Fig. 3j,k ) were similar to wild type. The organelles, however, remained distributed throughout the cytoplasm during meiosis II in all jas meiocytes ( Fig. 1n,r ; Supplementary Fig. 2j ). Following the chromosome separation in meiosis II, each group of chromosomes was incorporated into a new nucleus at telophase II ( Fig. 1u–x ). In jas meiocytes, the altered spindle position led to chromosome groups from different spindles being in close proximity to each other ( Fig. 1t , arrowhead; Supplementary Fig. 3e ), and two, three or four new nuclei were formed as co-located chromosome groups were incorporated into a common nucleus ( Fig. 1v,x ; Supplementary Fig. 3f,l ). At telophase II, the microtubules were reorganized into a radial array around each nucleus in wild type and jas , regardless of the nuclei number ( Fig. 1w,x ; Supplementary Fig. 3f,l ). The organelles were located between the nuclei and their associated radial microtubule arrays in both wild type and jas ( Fig. 1u,v ), suggesting that organelle positioning was not disturbed in jas at this stage. Following telophase II, cytokinesis occurs with a new cell wall being laid down where neighbouring radial microtubule arrays interact incorporating each nucleus into a single cell [17] , [18] , [19] . In wild type, this produced predominantly four-celled tetrads, while in jas a combination of tetrads (separated spindles), three-celled triads (tripolar-like spindles) and two-celled dyads (aligned spindles) were produced ( Fig. 2c ) as previously reported [11] , [12] . jas and ps1 meiocytes have distinct phenotypes Loss of PS1 also leads to a loss of spindle separation during meiosis II in A. thaliana [10] and it has been proposed that PS1 acts in a common genetic pathway with JAS [12] . We, therefore, examined whether PS1 also has a role in organelle positioning by examining DAPI-stained meiocytes maintained within the anther, similar to our analysis of jas . We did not examine microtubule location in ps1 as this had been reported prevously [10] . During the first meiotic division, organelles in ps1 remained clustered in regions of the cytoplasm close to the spindle, similar to the distribution in wild type and differing from the dispersed distribution observed in jas (compare Fig. 1a,b with Fig. 2d and Supplementary Fig. 2a–c ). Early in the second division, at prometaphase II, ps1 still appeared similar to wild type with well-separated chromosome groups ( Fig. 2a,e ) and the organelles predominantly located in the central organelle band ( Fig. 2e , arrow; Supplementary Fig. 2g ). As meiosis II progressed and cells entered metaphase II, the chromosome groups in most ps1 meiocytes were no longer fully separated ( Fig. 2b ). As the chromosome position reflects spindle position during meiosis II, it appears that disruption of spindle position was more severe in ps1 as there were more chromosome groups that were touching compared with jas ( Fig. 2b ). This difference in chromosome separation, and thus spindle separation in jas and ps1 , was reflected in different ratios of meiotic products with ps1 producing significantly more dyads than jas (58.5% vs 32.5%; χ 2 -test, P <10E−15) and jas producing significantly more triads than ps1 (43.4% vs 25.4%; χ 2 -test, P <10E−15; Fig. 2c ). By metaphase II, the organelle band had been lost in ps1 ( Fig. 2f ; Supplementary Fig. 2k ). Thus, ps1 appeared similar to jas at this stage, although loss of the organelle band occurred later. The differences in organelle distribution in meiosis I and early in meiosis II, along with the differences in the extent of spindle movement, reveal that jas and ps1 have distinct phenotypes. To determine whether these phenotypes were additive, we generated and analysed a jas ps1 double mutant. The organelle distribution in the double mutant was similar to that observed in the jas single mutant, with organelles distributed throughout the cytoplasm in meiosis I and meiosis II ( Fig. 2g–i ; Supplementary Fig. 2d,h,l ). Chromosome separation, and thus spindle position, was disturbed earlier in meiosis II in the double mutant than in either of the single mutants ( Fig. 2a ), and there were slightly more touching chromosome groups at metaphase II ( Fig. 2b ). Consistently, the proportion of dyads was significantly increased in the jas ps1 double mutant compared with jas and ps1 single mutants ( χ 2 -test, P <10E−15) with a corresponding decrease in the proportion of triads and tetrads ( Fig. 2c ). The increased disturbance in spindle position and the higher proportion of dyads in the jas ps1 double mutant is thus consistent with the jas and ps1 phenotypes being additive and reveal that JAS and PS1 act in separate genetic pathways. JAS co-localizes with markers for the endomembrane system To understand how JAS affects positioning of the organelles during meiosis, we investigated the subcellular localization of a JAS–GFP fusion protein under the control of the JAS promoter ( JAS:JAS–GFP ). This construct nearly completely complemented the jas phenotype with the majority of meiotic products being tetrads in three independent transgenic lines ( Supplementary Fig. 4 ). When viewed in meristematic roots cells, JAS–GFP was present in many subcellular compartments including the organelles and membranes ( Fig. 3b,f,j,n,r,v ). To gain insights into which the organelles and membranes of the cell JAS–GFP was localized to, we performed co-localization studies with a set of described endomembrane markers ( Fig. 3 ). A large fraction of the JAS–GFP-labelled organelles partially co-localized with Golgi ( Fig. 3a–d ) and trans-Golgi network ( Fig. 3e–h ) markers. JAS–GFP also showed some co-localization with a marker for the vacuolar membrane (the tonoplast; Fig. 3i–l ). There was also a weak GFP fluorescence associated with the plasma membrane, although there was not clear co-localization with the plasma membrane marker ( Fig. 3m–p ). On the other hand, JAS–GFP does not co-localize with markers for the peroxisome ( Fig. 3q–t ) or mitochondria ( Fig. 3u–x ). Overall, these data reveal that JAS is most likely associated with the endomembrane system potentially trafficking from the Golgi apparatus, through the trans-Golgi network, and to the tonoplast and plasma membranes in meristematic roots cells of A. thaliana . 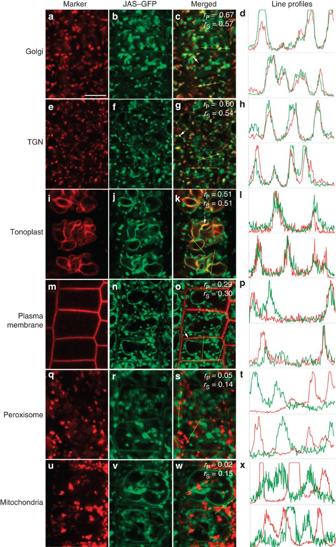Figure 3: JAS is located in the endomembrane system in roots. Roots from 4–6 day-old-A. thalianaseedlings expressing fluorescent fusion proteins that label the Golgi (a), the trans-Golgi network (TGN;e), the tonoplast (i), the plasma membrane (m) or the peroxisome (q) or stained with Mitotracker Red (u) and also expressingpJAS:JAS–GFP(b,f,j,n,r,v) were analysed by CLSM. The JAS–GFP pattern differs as images were taken at different focal planes to ensure that the labelled organelle (a,e,i,m,q,u) was in focus. For each marker, the red and green images were merged to assess co-localization (c,g,k,o,s,w). Co-localization is visualized by the presence of yellow in the merged images (examples are indicated with an arrow) and overlapping peaks of relative fluorescence intensity (yaxis) on lines that pass through areas with marker signal or staining (d,h,l,p,t,x). The position of the lines is indicated on the merged images and lines run from top to bottom or from left to right. Co-localization was also quantified by calculating the Pearson (rP) and Spearman (rS) correlation coefficients over the entire image except forowhere the plasma membrane regions were used. Values over 0.50 indicate co-localization. Scale bar, 10 μm. CLSM, confocal laser scanning microscopy. Figure 3: JAS is located in the endomembrane system in roots. Roots from 4–6 day-old- A. thaliana seedlings expressing fluorescent fusion proteins that label the Golgi ( a ), the trans-Golgi network (TGN; e ), the tonoplast ( i ), the plasma membrane ( m ) or the peroxisome ( q ) or stained with Mitotracker Red ( u ) and also expressing pJAS:JAS–GFP ( b , f , j , n , r , v ) were analysed by CLSM. The JAS–GFP pattern differs as images were taken at different focal planes to ensure that the labelled organelle ( a , e , i , m , q , u ) was in focus. For each marker, the red and green images were merged to assess co-localization ( c , g , k , o , s , w ). Co-localization is visualized by the presence of yellow in the merged images (examples are indicated with an arrow) and overlapping peaks of relative fluorescence intensity ( y axis) on lines that pass through areas with marker signal or staining ( d , h , l , p , t , x ). The position of the lines is indicated on the merged images and lines run from top to bottom or from left to right. Co-localization was also quantified by calculating the Pearson ( r P ) and Spearman ( r S ) correlation coefficients over the entire image except for o where the plasma membrane regions were used. Values over 0.50 indicate co-localization. Scale bar, 10 μm. CLSM, confocal laser scanning microscopy. Full size image As JAS acts during meiosis, we aimed at determining JAS localization in meiocytes ( Fig. 4 ). JAS–GFP was observed in the vicinity of the cluster of DAPI-stained organelles close to the spindle during meiosis I ( Fig. 4a–d ) and in the organelle band during meiosis II ( Fig. 4e–h ). Thus, JAS is located in the organelle cluster and organelle band consistent with its role in maintaining these structures. 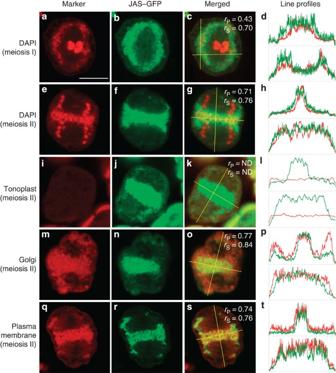Figure 4: In meiocytes JAS–GFP is located within the organelle cluster and organelle band and co-localizes with endomembrane markers. Meiocytes fromjasplants in meiosis I (a–d) or meiosis II (e–t), stained with DAPI (a,e) or expressing fluorescent fusion protein directed to the tonoplast (i), the Golgi apparatus (m) of the plasma membrane (q) and expressing eitherJAS:JAS–GFP(b,f,r) orUBQ14:JAS–GFP(j,n) were analysed by CLSM. For each marker, the red and green images were merged to assess co-localization (c,g,k,o,s). Co-localization is visualized by the presence of yellow in the merged images and overlapping peaks of relative fluorescence intensity on lines that pass through areas with marker signal or staining (d,h,l,p,t). The position of the lines is indicated on the merged images with the vertical line on top. Lines run from top to bottom or from left to right. Co-localization was also quantified by calculating the Pearson (rP) and Spearman (rS) correlation coefficients over entire meiocytes. Values over 0.50 indicate co-localization. Scale bar, 10 μm. CLSM, confocal laser scanning microscopy. Figure 4: In meiocytes JAS–GFP is located within the organelle cluster and organelle band and co-localizes with endomembrane markers. Meiocytes from jas plants in meiosis I ( a – d ) or meiosis II ( e – t ), stained with DAPI ( a , e ) or expressing fluorescent fusion protein directed to the tonoplast ( i ), the Golgi apparatus ( m ) of the plasma membrane ( q ) and expressing either JAS:JAS–GFP ( b , f , r ) or UBQ14:JAS–GFP ( j , n ) were analysed by CLSM. For each marker, the red and green images were merged to assess co-localization ( c , g , k , o , s ). Co-localization is visualized by the presence of yellow in the merged images and overlapping peaks of relative fluorescence intensity on lines that pass through areas with marker signal or staining ( d , h , l , p , t ). The position of the lines is indicated on the merged images with the vertical line on top. Lines run from top to bottom or from left to right. Co-localization was also quantified by calculating the Pearson ( r P ) and Spearman ( r S ) correlation coefficients over entire meiocytes. Values over 0.50 indicate co-localization. Scale bar, 10 μm. CLSM, confocal laser scanning microscopy. Full size image To identify which organelle(s) in the organelle band JAS is associated with, we used both JAS:JAS–GFP and a complementary DNA (cDNA) version of JAS expressed under the strong UBQ14 promoter ( UBQ14:JAS–GFP ), which also complemented the jas phenotype ( Supplementary Fig. 4 ). While both the DAPI-stained organelles and the JAS–GFP were present in the organelle band ( Fig. 4e,f ), they did not precisely overlap with the DAPI-stained organelles being confined to the central area of the region labelled by JAS–GFP ( Fig. 4g,h ). Given that JAS–GFP did not co-localize with the mitochondria in roots ( Fig. 3w,x ), and this difference in distribution within the organelle band, it is unlikely that JAS is localized to the mitochondria or plastids in meiocytes. As JAS was associated with the endomembrane system in roots, we investigated co-localization of JAS with markers of the tonoplast, Golgi apparatus and plasma membrane in JAS–GFP-containing meiocytes. The tonoplast marker produced a low signal that was most likely background, so co-localization of JAS–GFP with vacuole membranes could not be determined in meiocytes ( Fig. 4i–l ). Unlike the tonoplast marker, the Golgi marker was present in the organelle band but it had a wider distribution compared with the JAS–GFP signal being present in other regions of the meiocyte ( Fig. 4m,n ). Nevertheless, there was overlap of these markers within the organelle band ( Fig. 4o,p ), showing that JAS–GFP co-localized with a subset of the Golgi located in the organelle band during meiosis. The plasma membrane marker did not clearly label the plasma membrane in meiocytes, but instead was present in the organelle band ( Fig. 4q ). The plasma membrane marker is an aquaporin, and aquaporins have been reported to also localize to endomembrane vesicles [26] , [27] , [28] , [29] , [30] , making it likely that the signal is from endomembrane vesicles within the organelle band. JAS–GFP largely co-localized with this vesicle signal as both JAS–GFP and the plasma membrane maker were predominantly present in the organelle band, the width of the labelled region was similar and line profiles largely overlapped ( Fig. 4q–t ). Overall, we conclude that JAS is likely to be located in the endomembrane system in meiocytes, consistent with JAS localization in root cells, and is most likely associated with Golgi and endomembrane vesicles in the organelle band. In this study, we have used the jas mutant to reveal that organization of the cytoplasmic constituents is a critical aspect of plant meiosis. The most noticeable defect in jas meiocytes is the disruption of the relative position of the two spindles in the second meiotic division, and the resultant grouping of chromosomes from different spindles [12] ( Fig. 1 ). However, close examination of the jas phenotype indicates that the primary function of JAS is to maintain organelle position, as defects in organelle position occur in meiosis I and in meiosis II before there is any disturbance in spindle position. Furthermore, JAS is located in the organelle cluster and organelle band but is not directly associated with the spindle. This is consistent with spindle positioning defects being a consequence of altered organelle positioning and not being directly influenced by JAS. The distinct organization of organelles in the cytoplasm of plant cells undergoing male meiosis had previously been observed [17] , [18] , [19] , [20] , [21] , [22] , [23] , [24] , [25] , but little is known about their role or structure. We show that in A. thaliana , the organelles aggregate into a distinct cluster close to the spindle during meiosis I. A similar organelle clustering occurs in mouse oocytes with the mitochondria being perinuclear during meiosis I and II and it has been proposed that these aggregations ensure the provision of ATP for the energetically demanding processes involved in spindle formation and chromosome separation [31] , [32] . The clustering in plant meiocytes could serve similar functions or relate to processes of dedifferentiation, division and redifferentiation that these organelles pass through during meiosis [18] , [33] , [34] . The clustering at meiosis I is lost in jas meiocytes, showing that JAS is required for its presence. However, as the chromosomes behave in a similar manner and a functional bipolar spindle is formed in both wild-type and jas meiocytes, it does not appear to be essential for meiosis to progress. The second organelle aggregation that is lost in jas meiocytes is the organelle band that forms across the equator of cells at the end of meiosis I. This organelle band has been widely observed in plants [17] , [18] , [19] , [20] , [21] , [22] , [23] , [24] , [25] and its function has been speculated to relate to either the equal segregation of organelles into daughter cells at the end of meiosis or maintaining the physical separation of the two spindles during the second division. This work provides experimental data to distinguish these possibilities. Although the organelle band is lost during meiosis II in jas meiocytes, the organelle distribution during telophase II is similar to that observed in wild-type meiocytes ( Fig. 1 ), suggesting that the organelle band is unlikely to be required to ensure equal segregation of the organelles. Our data on the timing of events in jas meiocytes and JAS localization support the second possibility that the organelle band acts as a physical barrier. In jas meiocytes, the organelle band forms but is lost early in the second division before there is a decrease in spindle separation. This timing of events is consistent with the organelle band being required to maintain spindle separation rather than a pleiotropic effect where it would be expected that disturbances in the organelle band and spindle position would occur at the same time, or in a different order in different meiocytes. Furthermore, the presence of JAS specifically in the organelle band during meiosis II indicates that organelle band integrity, but not spindle position, is likely to be directly impacted on loss of JAS. We, therefore, propose that on loss of the organelle band in jas meiocytes, there is no longer a physical constraint and the spindles are free to move, and the degree of movement varies randomly between meiocytes. Some spindles display limited movement and remain separated, while others move more at one end producing the tripolar-like spindle structure, or move completely and become touching, parallel spindles. This produces the range of meiotic products (tetrads, triads and dyads) observed in the jas mutant [11] , [12] . Thus, our data support the idea that the organelle band is required to provide a physical barrier to prevent spindle interaction. The necessity of such a physical barrier is further supported from the analysis of meiosis in maize where cytokinesis normally occurs after the first meiotic division [35] . However, in maize mutants that fail to undergo this cytokinesis after meiosis I, there is no physical barrier separating the two spindles in meiosis II, and the spindles move closer together and form parallel and tripolar spindles similar to jas [35] . While the organelle band is likely to have an important role in separating the spindles, little is known about its structure. In most studies, the organelle band has been observed following staining of the DNA with DAPI, showing that it contains the mitochondria and/or plastids [17] , [18] , [19] , [20] , [21] , [22] , [23] , [24] , [25] . Our work reveals that a subset of the Golgi apparatus and endomembrane vesicles are also components of the organelle band. As these vesicles contain an aquaporin (PIP1;4) that is usually associated with the plasma membrane [26] , [36] , they may contain newly synthesized material that is destined to be transported to the plasma membrane. Alternatively, some of these vesicles could arise via endocytosis of the plasma membrane, as aquaporins are constitutively endocytosed and under certain conditions, including in mitosis, they can accumulate in intracellular vesicles [26] , [27] , [28] , [29] , [30] . The JAS protein co-localized with markers for the endomembrane system in roots and meiocytes, including the endomembrane vesicles that are part of the organelle band. We propose that it is these JAS-containing vesicles that are important for the maintenance of the organelle band. In mitotic cells, endomembrane vesicles are transported to the phragmoplast and contribute new membrane to the cell plate as it forms during cytokinesis [27] , [37] . We hypothesize that the JAS-containing vesicles in male meiocytes may be part of a similar process. While cytokinesis does not occur in many plant male meiocytes after the first division, early phragmoplast-like structures have been observed following meiosis I in a range of species [19] , [38] , [39] , indicating that the division process is initiated and then halted. Thus, in meiocytes, vesicles could be transported to the cell equator at the end of the first chromosome division, but no cell plate formation occurs. While these vesicles do not form a cell plate, our data show that they still play an important role as a physical barrier to maintain spindle separation, a process that relies on the associated JAS protein. Our analyses, furthermore, revealed that loss of a second protein, PS1, also known to impact on meiotic spindle position [10] results in a distinct phenotype compared with jas . In ps1 meiocytes, the organelle clustering is not disturbed in meiosis I and the organelle band in meiosis II is not completely lost until after chromosome positioning defects become apparent. Thus, unlike JAS, PS1 appears unlikely to have a primary role in controlling organelle position. These phenotypic differences on loss of JAS or PS1 function and the additive nature of the phenotypes suggest that they act in different genetic pathways to maintain spindle separation. Combined, our work highlights a thus far underappreciated role of endomembrane vesicles in plant meiosis and their impact on spindle positioning. We conclude that JAS is likely to be associated with endomembrane vesicles in meiocytes. These vesicles, through the action of the associated JAS protein, are required to maintain the physical structure of the organelle band, and thus keep the two spindles separated in the second meiotic division. Interestingly, a vesicle-based mechanism was recently reported to be important for the control of spindle position in animal meiocytes [40] . In mouse oocytes, the spindle must be positioned asymmetrically for the first meiotic division and vesicles are required for this spindle positioning. Hence, in both plants and animals, vesicles are important for correct spindle position in meiosis. Plant material Plants were grown in a growth room at 70% humidity and daily cycles of 16 h light and 8 h dark at 21 °C. The jas-1 allele in the Landsberg erecta accession [11] , the jas-3 allele (SAIL_813_H03) in the Columbia (Col) accession [11] and the ps1-1 allele (SALK_078818) in the Col accession [10] were as previously described. Transgenic lines were generated by Agrobacterium tumefaciens strain GV3101 mediated transformation using a standard floral dip method [41] . Fluorescent markers for the Golgi apparatus (SYP32-mCherry), the tonoplast (VAMP711-mCherry) and the plasma membrane (PIP1;4-mCherry) were from the wave line collection [36] , the trans-Golgi network marker was VHA-a1-mRFP [42] and the peroxisome marker was mRFP-PTS1 (ref. 43 ). Plasmid constructs To create pUBQ14:GFP–TUA6 , an expression cassette containing pNTM19:GFP–TUA6 in pGreen 0029 (ref. 44 ) was transferred into pPZP221 using XbaI and KpnI, and then ProNTM19 was replaced with a PCR-amplified pUBQ14 fragment (primers UBQ14F 5′–GTTATCTAGAATCCGAACAGAGTTAAACCGG-3′ and UBQ14R 5′–AATTCCCGGGAAACTGAGATTAATCGCTTGG-3′) using XbaI and SmaI. To create pJAS:JAS–GFP , a genomic fragment including the JAS promoter and genomic region without the stop codon was amplified (primers gJASF 5′-CACCGGATTAAGCTGTAACTGACCCGT-3′ and gJASR 5′-GAAGGAAACTACCGAGTTTGGT-3′) and subcloned into pENTR-D/TOPO. After sequencing, the genomic fragment was transferred into a modified form of pB7FWG2 (ref. 45 ) with the 35 S promoter removed. The pUBQ14:JAS–GFP construct was generated by Gateway multisite cloning (Invitrogen). DNA was amplified from genomic DNA ( pUBQ14 : primers as above) or cDNA ( JAS: primers cJASF 5′-ATGGCTTGTTTTCTCGACTGC-3′ and cJASR 5′-GAAGGAAACTACCGAGTTTG-3′) using Phusion high-fidelity polyermase (Finzymes) and primers with suitable attachment sites. PCR fragments were cloned into pDONR vectors and verified by sequencing. A multipart LR reaction using LR Clonase II plus and destination vectors pK7m34GW [46] was used to generate the expression vector. Microscopic and phenotypic analyses To test for complementation and analysis of meiocytes maintained in the anther, inflorescences were harvested and fixed overnight in 3:1 ethanol:acetic acid. Buds were then separated and anthers containing meiocytes were dissected. Anthers were either dissected to release meiocytes (complementation analysis) or placed directly on a microscope slide. Material was then stained with DAPI (0.4 mg ml −1 ) in phosphate buffer (100 mM sodium phosphate (pH 7.0), 1 mM EDTA and 0.1% Triton X-100) for 5 min, covered and viewed directly. The distance between the chromosome groups was measured in ImageJ on single optical sections where both the chromosome groups were clearly visible. For GFP localization studies in meiocytes whole inflorescences from plants containing pUBQ14:GFP–TUA6 , pJAS:JAS–GFP or pUBQ14:JAS–GFP were fixed in 100% methanol for 20 min at −20 °C and washed with phosphate-buffered saline, pH 7.4 at 4 °C. Anthers containing meiocytes were dissected from floral buds and gently torn open using fine needles. Material was then stained with DAPI (as above) to allow meiotic stages to be determined and viewed. For observing roots, seedlings were germinated for 4–6 days on ½ strength Murashige and Skoog agar. Fluorescent protein fusions were observed in roots mounted in water and roots were stained with 500 nM Mitotracker Red (Molecular Probes) for 5 min, washed and mounted in water. Images were taken at different focal planes such that the labelled organelle or membrane was in focus. Counting of meiotic products was performed under a Leica DMIRE2 inverted microscope. All confocal images were taken using a Leica SP2-AOBS Point Laser Scanning Confocal Microscope or a Zeiss 780 Confocal Laser Scanning Microscope. The following excitation and detection wavelengths were used: DAPI 405 nm excitation, 415–470 nm detection; GFP 488 nm excitation, 500–550 nm detection; mCherry/mRFP/Mitotracker Red 561 nm excitation 580–650 nm detection. Images were captured using the Imaris software (Version 7.1.x) and manipulated using ImageJ and Photoshop. Pearson and Spearman correlation coefficients were calculated using the PSC co-localization plugin in Image J [47] with the background intensity noise threshold set to zero. For root images, the whole image was used, expect for the plasma membrane marker where only the region containing the plasma membrane was used due to the weak nature of the GFP signal in the plasma membrane compared with other organelles. For meiocytes, only the region of the image containing the meiocytes was used. Line profiles were performed on overlay images using the RGBProfiles Tool in ImageJ and data processed in Excel. To directly compare relative fluorescence levels in the different colour channels, the fluorescence for each line was normalized such that the highest level was set to a value of one. This was conducted for all profiles except for those in Fig. 4l where the red fluorescence in a neighbouring non-meiocytes cell was set to one, due to the low level of signal in meiocytes. How to cite this article: Brownfield, L. et al . Organelles maintain spindle position in plant meiosis. Nat. Commun . 6:6492 doi: 10.1038/ncomms7492 (2015).